A single locus confers tolerance to continuous light and allows substantial yield increase in tomato An important constraint for plant biomass production is the natural day length. Artificial light allows for longer photoperiods, but tomato plants develop a detrimental leaf injury when grown under continuous light—a still poorly understood phenomenon discovered in the 1920s. Here, we report a dominant locus on chromosome 7 of wild tomato species that confers continuous light tolerance. Genetic evidence, RNAseq data, silencing experiments and sequence analysis all point to the type III light harvesting chlorophyll a/b binding protein 13 ( CAB-13 ) gene as a major factor responsible for the tolerance. In Arabidopsis thaliana , this protein is thought to have a regulatory role balancing light harvesting by photosystems I and II. Introgressing the tolerance into modern tomato hybrid lines, results in up to 20% yield increase, showing that limitations for crop productivity, caused by the adaptation of plants to the terrestrial 24-h day/night cycle, can be overcome. Experiments in the 1920s revealed that tomato ( Solanum lycopersicum ) plants, when grown under continuous light (CL), develop a potentially lethal injury characterized by mottled leaf chlorosis and necrosis [1] . However, many other plant species, like the model plant Arabidopsis ( Arabidopsis thaliana ) [2] , [3] , pepper ( Capsicum annuum ) [4] , [5] , [6] , [7] , [8] , lettuce ( Lactuca sativa ) [1] , [9] and rose ( Rosa x hybrida ) [10] , [11] are not injured by CL. 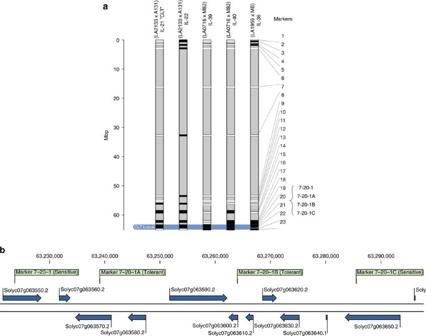Figure 1: Chromosomal localization of CL tolerance. (a) The CL tolerance locus is located in the lower arm of chromosome seven (grey columns). Based on the public tomato reference genome v2.40 (ref.24), SNP markers positions are in Mpb. White horizontal bars representS. lycopersicumalleles, and black bars represent non-S. lycopersicumalleles in several CL-tolerant IL (see accession number of each parent at the top). All alleles are homozygous for either parent. According to 361 additional markers, the other eleven chromosomes are homozygous forS. lycopersicum(with the exception of two markers in some lines; these exceptions have no relevance for the CL tolerance localization). All non-S. lycopersicumparents are CL tolerant; hence, the CLT locus was initially mapped between markers 19 and 22 (1.2 Mbp) and represented by a horizontal blue bar. From the LA2133 × A131 population, IL-21 is named ‘CLT’ and used for further research in this study. (b) After fine mapping CL tolerance in ‘CLT’ F3families, the locus was further located between markers 7-20-1A and 7-20-1B, which segregated as tolerant in the F3. Markers 7-20-1 and 7-20-1C segregated as sensitive in the F3. TheCAB-13gene (Solyc07g063600.2) contains the marker 7-20-1B, which is associated with CL tolerance, and its role in the CL tolerance was further tested in this study. Hence, the high sensitivity to CL of tomato, an emerging model organism for the Solanaceae family and fleshy fruited plants [12] , is intriguing and has motivated plenty of research efforts (see Supplementary Table 1 for complete literature list and for reviews see refs 13 , 14 , 15 ). More than eight decades after the original discovery, however, the physiological basis of this CL-induced injury remains poorly understood. In contrast to natural day/night cycles, CL implies continuous energy supply for photosynthesis, continuous photooxidative pressure, continuous signalling to the photoreceptors and a mismatch between the internal circadian clock frequency and the external light/dark cycle known as circadian asynchrony [13] . The importance of these four components on the CL-induced injury has been previously investigated in several experimental setups. For instance, carbohydrate accumulation, which presumably results from continuous energy supply for photosynthesis, has been regarded for a long time as a potential trigger of CL-induced injury [1] , [7] , [13] , [16] . The photoinhibition and adaptation of photosystems I and II (PSI and PSII) have been studied in CL-grown tomatoes by ref. 8 . Addition of far-red light to the CL treatment reduced injury symptoms [17] , suggesting an involvement of phytochromes. Finally, the role of circadian asynchrony on the CL-induced injury has been examined and/or suggested in several papers [13] , [18] , [19] , [20] , [21] . However, concluding which component induces the injury is not simple because, in most cases, CL affects all four components simultaneously. We have proposed that a combination of these components could induce the injury rather than a particular one on its own [13] . Understanding why CL injures tomato plants is not only valuable for fundamental research but also has potential applications, as tomato is the most important vegetable crop worldwide. Under greenhouse conditions, a tomato crop simulation model, TOMSIM [22] , predicted that a hypothetical CL-tolerant tomato genotype, would yield between 22 and 26% more fruits when using supplementary lighting for 24 h per day (CL) in comparison with using supplementary lighting only for 18 h per day during daytime under Dutch greenhouse conditions [23] . In this study, we locate CL tolerance, mapping to the lower arm of chromosome 7, in eight wild tomato accessions. Genetic evidence, RNAseq data, silencing experiments and sequence analysis all point to the type III Light Harvesting Chlorophyll a/b Binding protein 13 ( CAB-13 ) gene as a major factor responsible for the tolerance. By introgressing the tolerance into modern tomato F 1 hybrid lines, we achieve up to a 20% yield increase. This not only proves that limitations for crop productivity, caused by the adaptation of plants to the terrestrial 24-h day/night cycle, can be overcome but also opens new research lines in the most important process of photosynthesis. CL tolerance across the Solanum genus Looking for CL tolerance, we exposed nine wild tomato accessions to CL. All but one wild tomato accessions ( Solanum pimpinellifolium LA1589) were CL tolerant ( Supplementary Table 1 ). We also tested several S. lycopersicum genotypes including reference lines (Heinz, Moneyberg, Moneymaker and M82), a modern inbred line (A131), F 1 hybrid cultivars (for example, Encore, Tourance and Westland), rootstocks (for example, Maxifort) and an heirloom variety (Sub-Arctic Plenty); all genotypes but one (Sub-Arctic Plenty) were CL sensitive ( Supplementary Table 1 ). From literature, we collected phenotypic data of additional wild tomato species, inter-species hybrids, modern F 1 hybrid tomato cultivars, heirloom tomato varieties and related species like potato ( Solanum tuberosum ) and eggplant ( Solanum melongena ). The occurrence of CL tolerance and sensitivity across the Solanum genus facilitates physiological and genetic studies on this trait. CL tolerance is a dominant trait We used 96 introgression lines (IL) from three populations, genotyped with 384 single-nucleotide polymorphism (SNP) markers, to map the CL tolerance. All lines carrying an introgression in the lower arm of chromosome 7, derived from a CL-tolerant wild donor, were CL tolerant ( Supplementary Table 1 ). CL tolerance was initially mapped between SNP markers 19 and 22 ( Fig. 1a ). To investigate the inheritance of the trait, CL-tolerant IL-21 (here after named ‘CLT’) and 22, both from the LA2133 × A131 population, were crossed with their recurrent CL-sensitive parent (A131). F 1 progeny were all CL tolerant, indicating that the trait is dominant. F 1 plants were self-fertilized to produce an F 2 generation; when 769 plants were exposed to CL, they segregated 2.95:1.05 tolerant:sensitive (568 tolerant:201 sensitive, X 2 [3:1]=0.53; P =0.47). This strongly suggests that CL tolerance is a monogenic, dominant trait. Using F 2 plants with a recombination between markers 19 and 22, 18 F 3 families were generated. After genotyping with additional SNP markers, the plants were exposed to CL, and the CL tolerance locus was fine-mapped between markers 7-20-1A and 7-20-1B. The physical distance between these markers is ~25 kb, and only four genes are located between them; when identifying the gene responsible for the CL tolerance, additional genes in the vicinity were considered ( Fig. 1b ). Figure 1: Chromosomal localization of CL tolerance. ( a ) The CL tolerance locus is located in the lower arm of chromosome seven (grey columns). Based on the public tomato reference genome v2.40 (ref. 24 ), SNP markers positions are in Mpb. White horizontal bars represent S. lycopersicum alleles, and black bars represent non- S. lycopersicum alleles in several CL-tolerant IL (see accession number of each parent at the top). All alleles are homozygous for either parent. According to 361 additional markers, the other eleven chromosomes are homozygous for S. lycopersicum (with the exception of two markers in some lines; these exceptions have no relevance for the CL tolerance localization). All non- S. lycopersicum parents are CL tolerant; hence, the CLT locus was initially mapped between markers 19 and 22 (1.2 Mbp) and represented by a horizontal blue bar. From the LA2133 × A131 population, IL-21 is named ‘CLT’ and used for further research in this study. ( b ) After fine mapping CL tolerance in ‘CLT’ F 3 families, the locus was further located between markers 7-20-1A and 7-20-1B, which segregated as tolerant in the F 3 . Markers 7-20-1 and 7-20-1C segregated as sensitive in the F 3 . The CAB-13 gene (Solyc07g063600.2) contains the marker 7-20-1B, which is associated with CL tolerance, and its role in the CL tolerance was further tested in this study. 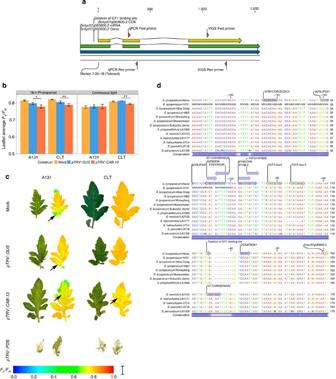Figure 2:CAB-13is involved in CL tolerance in tomato. (a) Structure of the tomatoCAB-13gene on chromosome 7, consisting of three exons. The mRNA is depicted with green arrows and the coding region with yellow arrows. Red arrows indicate the primers used for VIGS and RT–qPCR. A molecular marker associated with CL tolerance is also indicated. (b) Maximum efficiency of PSII (Fv/Fm) of A131 and CLT plants treated with severalpTRVconstructs before (left panel, 16-h photoperiod) and after exposure to CL (right panel, CL). Values represent mean±s.e.m.,n=4 plants. Asterisks represent statistical difference betweenpTRV::GUSandpTRV::CAB-13(other contrasts are not presented); *P<0.05, **P<0.01, Fisher’s protected LSD test. Scale bar, 2 cm. (c) CL-induced injury in Mock,pTRV::GUS,pTRV::CAB-13andpTRV::PDS-treated A131 and CLT plants as seen by RGB images (left) and chlorophyll fluorescence images (right). Notice the characteristic mottled chlorosis induced by CL (indicated with arrows). (d) Promoter region ofCAB-13of several CL-sensitive and -tolerant lines. Predicted regulatory elements are highlighted with blue and green arrows (seeSupplementary Table 4for the complete list). Notice the 9-pb deletion of GT-1 binding site shared by all CL sensitive lines (with the exception of Sub-Arctic Plenty). Full size image After pooling publicly available tomato and wild tomato genome sequences [24] , [25] and RNAseq-derived transcriptomes (details below), we compared the sequence of all genes in the CL tolerance locus vicinity belonging to five CL-tolerant and five CL-sensitive genotypes ( Supplementary Table 2 ). 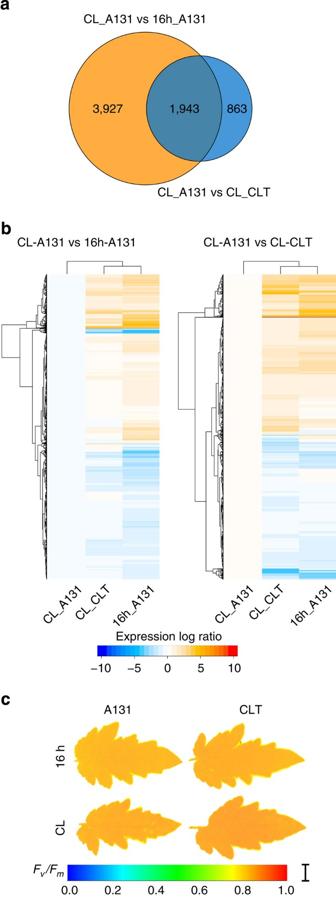Figure 3: RNAseq analysis. (a) Venn diagram showing the number of differentially regulated genes between A131 exposed to 16-h photoperiod and CL (left, orange) and between A131 and CLT exposed to CL (right, blue). (b) Hierarchical clustering of differentially regulated genes. A single coloured horizontal line represents each gene. The colours represent the relative expression level of that gene,n=3. (c) Chlorophyll fluorescence images of representative leaves used in the experiment. Scale bar, 2 cm. In addition, Supplementary Table 3 shows the expression of all genes in the CL tolerance locus evaluated with RNAseq. From all genes in the locus, the type III Light harvesting chlorophyll a/b binding protein 13 gene ( LHCB type III CAB-13 or CAB-13, Solyc07g063600.2 ) is the most likely candidate to confer tolerance to CL, as it was downregulated when exposed to CL in A131 plants, a 9-base deletion was detected in its promoter region in all CL-sensitive lines and it is known to be involved in light harvesting for photosynthesis ( Supplementary Tables 2 and 3 ). CAB-13 silencing impairs CL tolerance To confirm that CAB-13 is responsible for the CL tolerance in tomato, we silenced its expression in a CL-tolerant line (CLT) using virus-induced gene silencing (VIGS). The chlorophyll fluorescence parameter F v /F m , which is widely used to assess biotic and abiotic stress [26] , was selected to quantify the level of CL-induced injury. The parameter F v /F m represents the maximum quantum efficiency of PSII; therefore, the lower the F v /F m value, the higher the injury is. The tomato CAB-13 gene consists of three exons; a unique region from exon 3 was cloned into the VIGS vector pTRV [27] , [28] ( Fig. 2a ). The pTRV::PDS [27] and pTRV::GUS [29] constructs were used as positive and negative controls, respectively. Figure 2: CAB-13 is involved in CL tolerance in tomato. ( a ) Structure of the tomato CAB-13 gene on chromosome 7, consisting of three exons. The mRNA is depicted with green arrows and the coding region with yellow arrows. Red arrows indicate the primers used for VIGS and RT–qPCR. A molecular marker associated with CL tolerance is also indicated. ( b ) Maximum efficiency of PSII ( F v /F m ) of A131 and CLT plants treated with several pTRV constructs before (left panel, 16-h photoperiod) and after exposure to CL (right panel, CL). Values represent mean±s.e.m., n =4 plants. Asterisks represent statistical difference between pTRV::GUS and pTRV::CAB-13 (other contrasts are not presented); * P <0.05, ** P <0.01, Fisher’s protected LSD test. Scale bar, 2 cm. ( c ) CL-induced injury in Mock, pTRV::GUS , pTRV::CAB-13 and pTRV::PDS -treated A131 and CLT plants as seen by RGB images (left) and chlorophyll fluorescence images (right). Notice the characteristic mottled chlorosis induced by CL (indicated with arrows). ( d ) Promoter region of CAB-13 of several CL-sensitive and -tolerant lines. 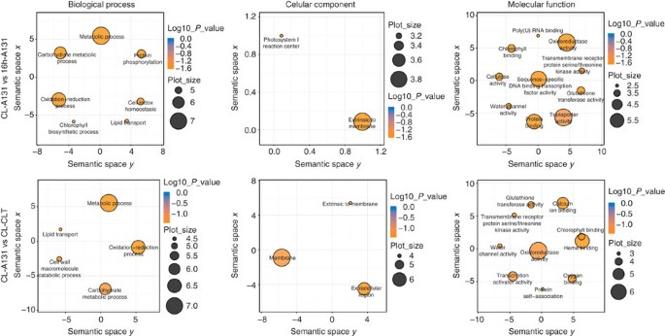Figure 4: GO enrichment analysis. GO terms significantly enriched for two contrast (see labels at the left) and three GO categories (see labels at the top). Each circle represents a GO term. Within the Cartesian coordinates (x,y), the closer the circles rest, the more related the GO terms are. The size of the circles is proportional to the number of child GO terms. The circle colour represents the significance of the enrichment. Predicted regulatory elements are highlighted with blue and green arrows (see Supplementary Table 4 for the complete list). Notice the 9-pb deletion of GT-1 binding site shared by all CL sensitive lines (with the exception of Sub-Arctic Plenty). Full size image Regardless of the tomato genotype, all pTRV::PDS -infiltrated plants showed photobleaching symptoms ( Supplementary Fig. 1 ), indicating that pTRV infection efficiency was close to, or even at, 100%. As expected [27] , the occurrence of photobleached spots within these plants was patchy ( Supplementary Fig. 1a ). Therefore, the reverse transcriptase quantitative PCR (RT–qPCR) data of all pTRV-infected plants ( Supplementary Fig. 1b ) should be taken with caution as, unlike chlorophyll fluorescence imaging, only a small leaf area was sampled. Under 16-h photoperiod, CLT and control A131 plants infiltrated with pTRV::CAB-13 showed slightly lower F v /F m than control plants infiltrated with pTRV:GUS ( Fig. 2b ), yet no chlorosis was observed. After 3 weeks of CL, the F v /F m was low in all A131 plants regardless of the VIGS construct, but CLT plants kept a high F v /F m with the exception of pTRV::CAB-13 infiltrated plants ( Fig. 2b ). In addition to the low F v /F m , these plants showed interveinal chlorosis characteristic of the CL-induced injury ( Fig. 2c ). Considering that (i) the leaf area imaged with the chlorophyll fluorescence camera was much larger than the leaf area harvested for qPCR and that (ii) the appearance (at the expected time and in the expected leaves) of the characteristic CL-induced interveinal chlorosis in CL-tolerant plants after exposure to CL unequivocally indicates that the tolerance has been broken, the results show that CAB-13 plays a key role in the CL tolerance in tomato. A deletion in CAB-13 is present in all sensitive lines To further investigate the role of CAB-13 in the CL tolerance, the PlantPAN [30] tool was used to identify regulatory elements in the promoter region. Among others, tomato CAB-13 promoter contains putative regulatory elements associated to light-responsive, photosynthetic and circadian clock-controlled genes like GT-1 consensus [31] , SORLIP2AT [32] , −10PEHVPSBD [33] , GATA box [34] and the EVENINGAT [35] ; all identified putative regulatory elements are summarized in Supplementary Table 4 . Remarkably, one of these regulatory elements, the second copy of GT-1 consensus, is deleted in all CL-sensitive lines ( Fig. 2d ), suggesting that GT-1 transcription factor is involved in the CL tolerance/sensitivity in tomato. Interestingly, Sub-Arctic Plenty cultivar also has a deletion of GT-1 consensus, comparable with sensitive cultivars ( Fig. 2d ), yet they are CL tolerant ( Supplementary Table 1 ). We were not able to find in literature a described cross with a CL-tolerant wild tomato in its lineage [36] , [37] . Therefore, a CAB-13 -independent CL tolerance in Sub-Arctic Plenty cannot be ruled out. Considering that Sub-Arctic Plenty tomato cultivar was bred in the most northern agricultural research establishment in Canada (The Beaverlodge Research Farm, http://www4.agr.gc.ca ) [37] , an unintended selection for CL tolerance, driven by long summer days, is a possibility. Disruption of carbohydrate metabolism and photosynthesis To identify metabolic pathways altered by CL in uninjured leaves, we performed gene expression analysis and gene ontology (GO) enrichment analysis on RNAseq-derived data. First, we identified differentially expressed genes in the contrasts CL A131 versus 16 h A131 and CL A131 versus CL CLT ( Fig. 3 and Supplementary Tables 5 and 6 ). The first contrast evaluates the effect of CL in A131 plants, and the second one evaluates the genotype effect under CL. From the 31,350 genes that passed quality control, we found 5,870 and 2,806 differentially expressed genes in response to CL and genotype, respectively ( Fig. 3a ); Fig. 3b shows cluster analyses for each contrast. The number of genes differentially regulated in both contrasts was 1,943; hence, the differentially regulated genes that responded exclusively to CL or genotype were 3,927 and 863, respectively. In the GO enrichment analysis, 19 and 17 GO terms were found significantly enriched for each contrast. Data are summarized in Fig. 4 ; the closer two given terms lie in the semantic space [38] ( x and y coordinates), the more similar they are. In addition, the size of each GO term indicates how general it is, and the colour indicates the significance of enrichment ( Fig. 4 ). Among others, the GO terms ‘carbohydrate metabolic process’, ‘chlorophyll biosynthetic process’, ‘photosystem I reaction centre’ and ‘chlorophyll binding’ were enriched when A131 plants are exposed to CL. Similarly, the terms ‘carbohydrate metabolic process’, ‘chlorophyll binding’ and ‘heme binding’ were enriched in CLT as compared with A131 when exposed to CL. These results indicate that photosynthesis and carbohydrate metabolism are strongly affected by CL at the transcriptional level, even in adult, uninjured leaves ( Fig. 3c ). Figure 3: RNAseq analysis. ( a ) Venn diagram showing the number of differentially regulated genes between A131 exposed to 16-h photoperiod and CL (left, orange) and between A131 and CLT exposed to CL (right, blue). ( b ) Hierarchical clustering of differentially regulated genes. A single coloured horizontal line represents each gene. The colours represent the relative expression level of that gene, n =3. ( c ) Chlorophyll fluorescence images of representative leaves used in the experiment. Scale bar, 2 cm. Full size image Figure 4: GO enrichment analysis. GO terms significantly enriched for two contrast (see labels at the left) and three GO categories (see labels at the top). Each circle represents a GO term. Within the Cartesian coordinates ( x , y ), the closer the circles rest, the more related the GO terms are. The size of the circles is proportional to the number of child GO terms. The circle colour represents the significance of the enrichment. Full size image Development is not affected in tolerant lines Parallel to our genetic and physiological work, we also developed and tested an application of the CL tolerance. After years of breeding (up to six generations), F 1 hybrid lines, tolerant to CL, in the background of elite commercial cultivars (Idooll and Westland) were used in a yield trial in the 2012–2013 winter season. Pilot trials done in previous years showed that compensation measures were needed for the extra assimilates available under CL. Therefore, crop density was increased, CL was applied gradually only starting after the crop became generative ( Fig. 5a ) and the temperature was managed according to each treatment needs. The resulting climate conditions within the greenhouse are reported in Supplementary Fig. 2 . 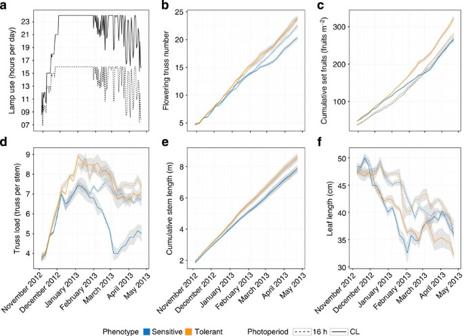Figure 5: Developmental measurements during the yield trial. Measurements were done on Idooll F1CL-tolerant and -sensitive homozygous lines; parent lines where backcrossed four times with a CL-tolerant introgression line, beingSolanum pennelliithe wild donor. (a) Hours a day that the lamps where on. Between November and December, the photoperiod set point was increased in 4 and 5 steps from 10 and 12 to 16 and 24 h per day, respectively. During the dark winter months of December and January, the lamps are on during the complete ‘light’ period. Later during the season, however, solar irradiance was, at times, high (>350 W m−2) so lamp use was not needed during some hours a day to achieve the set point of 16 and 24 h of light per day. (b) Flowering truss number. (c) Cumulative set fruits. (d) Number of fruits per stem. Around February, the CL-sensitive tomato plants exposed to CL became so sick, that we were forced to prune trusses in order to save the plants and keep the trial going. (e) Cumulative stem length. (f) Length of the topmost fully expanded leaf. (b–f) Measurements were done weekly, values are mean±s.e.m. (grey shadow),n=4. Figure 5: Developmental measurements during the yield trial. Measurements were done on Idooll F 1 CL-tolerant and -sensitive homozygous lines; parent lines where backcrossed four times with a CL-tolerant introgression line, being Solanum pennellii the wild donor. ( a ) Hours a day that the lamps where on. Between November and December, the photoperiod set point was increased in 4 and 5 steps from 10 and 12 to 16 and 24 h per day, respectively. During the dark winter months of December and January, the lamps are on during the complete ‘light’ period. Later during the season, however, solar irradiance was, at times, high (>350 W m −2 ) so lamp use was not needed during some hours a day to achieve the set point of 16 and 24 h of light per day. ( b ) Flowering truss number. ( c ) Cumulative set fruits. ( d ) Number of fruits per stem. Around February, the CL-sensitive tomato plants exposed to CL became so sick, that we were forced to prune trusses in order to save the plants and keep the trial going. ( e ) Cumulative stem length. ( f ) Length of the topmost fully expanded leaf. ( b – f ) Measurements were done weekly, values are mean±s.e.m. (grey shadow), n =4. Full size image To better understand how CL affects development and ecology of the crop in the long term, we took weekly measurements of key parameters that, if affected, could have an impact on yield ( Fig. 5 ). No difference was found in flowering truss appearance rate between CL-tolerant plants cultivated under 16-h photoperiod and CL ( Fig. 5b ). Considering that average daily temperature was similar in both photoperiods ( Supplementary Fig. 2c ), these results indicate that CL does not have an effect on development rate in tomato. Similarly, we found no effect of CL on fruit set in CL-tolerant plants ( Fig. 5c ). In CL-sensitive plants, in contrast, CL injured the plants so badly that development and fruit set were severely reduced ( Fig. 5b,c ). Around February, actually, trusses from CL-sensitive plants cultivated under CL were pruned in order to rescue the plants and to proceed with the experiment—a dead plant within the crop would mean a disruption in the canopy structure that could compromise the validity of the trial. Figure 5d shows the resulting truss load. Regardless of the light treatment, flowers opened only during daytime and closed during the night or subjective night. This indicates that the circadian clock was still running in the plants and was probably reset by daily changes in temperature and light. Given that bumblebees were only allowed to exit the hive between sunrise and sunset, we encountered no problems with pollination. As seen in Fig. 5e , CL had no effect on stem elongation, but the CLT was longer than the CL-sensitive line. To avoid differences in light interception by the different lines, we kept the top of each plant at the same height. CL-exposed tomato leaves tend to have smaller leaf area [20] . The weekly leaf length measurements ( Fig. 5f ) showed shorter leaves. The visibly open canopy observed in the CL-grown crop most likely resulted from a lower leaf area. Photosynthesis during CL in tomato To know whether CL-tolerant plants can use the artificial light provided during night to efficiently fix carbon, we measured photosynthetic gas exchange every minute during 2 days and nights using ambient light. Regardless of the photoperiod, photosynthesis rate closely correlated with light intensity ( Supplementary Fig. 3a,b ). We found no difference in the quantum efficiency of CO 2 fixation (ΦCO 2 ) between day and night in CL-cultivated plants ( Supplementary Fig. 3c ), indicating that CL-tolerant plants are able to use the artificial light provided at night to efficiently fix CO 2 . To assess the effects of CL on photosynthesis in more detail, we performed photosynthesis measurements using combined gas exchange and chlorophyll fluorescence techniques. In representative leaves of each genotype and light treatment, leaf absorbance across the photosynthetically active spectrum was measured ( Fig. 6a ) and later used in computation of several parameters. As expected, CL-injured leaves had a lower leaf absorbance as the result of chlorosis. Light and CO 2 response curves showed that photosynthesis greatly diminished in CL-sensitive tomatoes when grown under CL ( Fig. 6b,c ). In contrast, CL-tolerant leaves only showed a slight decrease in photosynthesis rate across light and CO 2 levels. This decrease could not be attributed to a single aspect of the photosynthetic machinery as most of the estimated parameters of the Farquhar-von Caemmerer-Berry (FvCB) [39] model were slightly diminished in CL-tolerant tomatoes when grown under CL ( Table 1 ). 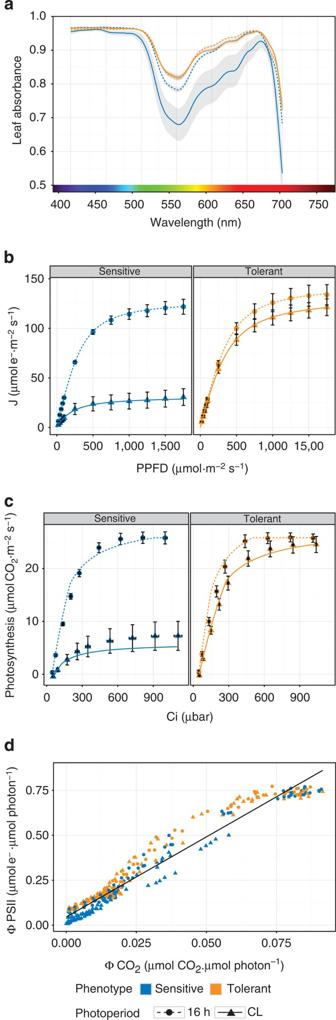Figure 6: Photosynthetic responses of tomato leaves to CL. (a) Absorbance of CL-tolerant and -sensitive leaves developed under 16-h photoperiod or CL. Mean±s.e.m. (grey shadow),n=3. (b) Response of J (electron transport) to light (PPFD). Mean±s.e.m.,n=4. Lines were drawn by fitting the predicted parameters (Table 1) to the FvCB model. (c) Response of photosynthesis to intracellular CO2concentration (Ci). Mean±s.e.m.,n=4 leaves. Lines were drawn by fitting the predicted parameters (Table 1) to the FvCB model. (d) Relationship between the quantum efficiency of PSII e−flow on PSII-absorbed light basis (ΦPSII) and the quantum efficiency of CO2assimilation on the leaf PPFD-absorbed basis (ΦCO2) in CL-tolerant and -sensitive leaves developed under 16-h photoperiod or CL. Figure 6d shows the relation between the quantum efficiency of PSII e − flow (ΦPSII) and the quantum efficiency of CO 2 assimilation (ΦCO 2 ). The data fitted well to the FvCB model as indicated by high r 2 values (>0.98); although this was not the case for data from CL-sensitive leaves exposed to CL ( Table 1 ), photosynthetic parameters estimated from these leaves should be taken with caution as a large variation from leaf to leaf was observed in CL-injured leaves. Figure 6: Photosynthetic responses of tomato leaves to CL. ( a ) Absorbance of CL-tolerant and -sensitive leaves developed under 16-h photoperiod or CL. Mean±s.e.m. (grey shadow), n =3. ( b ) Response of J (electron transport) to light (PPFD). Mean±s.e.m., n =4. Lines were drawn by fitting the predicted parameters ( Table 1 ) to the FvCB model. ( c ) Response of photosynthesis to intracellular CO 2 concentration (Ci). Mean±s.e.m., n =4 leaves. Lines were drawn by fitting the predicted parameters ( Table 1 ) to the FvCB model. ( d ) Relationship between the quantum efficiency of PSII e − flow on PSII-absorbed light basis (ΦPSII) and the quantum efficiency of CO 2 assimilation on the leaf PPFD-absorbed basis (ΦCO 2 ) in CL-tolerant and -sensitive leaves developed under 16-h photoperiod or CL. Full size image Table 1 Photosynthetic parameters of CL-tolerant and -sensitive tomato leaves developed under 16-h photoperiod or CL. Full size table CL can increase tomato yield As expected, most CL-sensitive tomato lines yielded less kilograms of tomatoes per m 2 when grown under CL as compared with 16-h photoperiod ( Fig. 7 ). In contrast, continuous light tolerant lines produced the same or more tomatoes under CL than under 16-h photoperiod. The yield increase was up to 20% in the line with the highest number of backcrosses (CL-tolerant homozygous, Idooll_pen5940). Even though some continuous light tolerant lines did not show significant yield increase at the end of the trial (April 2013, Fig. 7 ), they did show a trend to yield more under CL than 16-h photoperiod up to mid March 2013 ( Supplementary Fig. 4 ). Considering that most of the lines showing significant yield increase under CL were heterozygous for CL tolerance, a potential linkage drag could explain why no clear trend in tomato yield was observed when comparing the CL-sensitive lines cultivated under 16-h photoperiod with the continuous light tolerant lines cultivated under CL. Remarkably, a heterozygous continuous light tolerant line cultivated under CL achieved the highest yield (21.4 kg m −2 ). 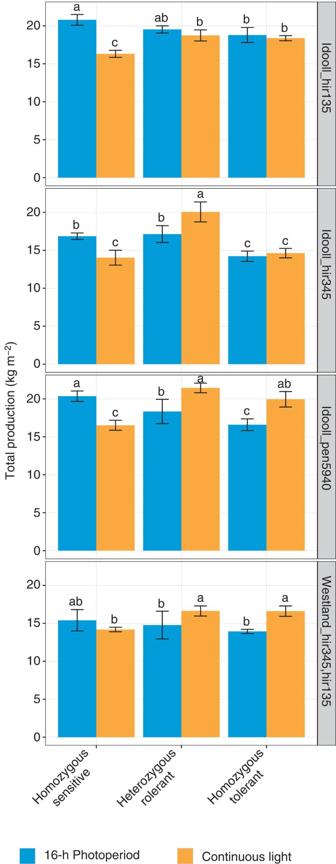Figure 7: Yield under 16-h photoperiod and CL. Each panel depicts the yield of F1hybrids grouped in four categories; in each category, several CL-tolerant IL were backcrossed with the parents of ‘Idooll’ or ‘Westland’ F1commercial hybrids (see background and wild donor on the right). After 3–4 backcrosses, the newly bread parents, segregating as CL-tolerant or -sensitive, were used to generate homozygous or heterozygous and tolerant or sensitive Idooll and Westland F1hybrids (see labels at the bottom). Mean±s.e.m.,n=3 plots. Within each of the four groups, bars with different letter are statistically different (P<0.05), Fisher’s protected LSD test. Figure 7: Yield under 16-h photoperiod and CL. Each panel depicts the yield of F 1 hybrids grouped in four categories; in each category, several CL-tolerant IL were backcrossed with the parents of ‘Idooll’ or ‘Westland’ F 1 commercial hybrids (see background and wild donor on the right). After 3–4 backcrosses, the newly bread parents, segregating as CL-tolerant or -sensitive, were used to generate homozygous or heterozygous and tolerant or sensitive Idooll and Westland F 1 hybrids (see labels at the bottom). Mean±s.e.m., n =3 plots. Within each of the four groups, bars with different letter are statistically different ( P <0.05), Fisher’s protected LSD test. Full size image It is well known that domesticated tomatoes are sensitive to CL; interestingly, S. pimpinellifolium , the closest relative of domesticated tomatoes [24] , is CL sensitive too ( Supplementary Table 1 ). In contrast, all other tested wild tomatoes are tolerant to CL. This suggests that this trait was lost during domestication. Whether tolerance to CL provides an adaptive advantage in nature is not known since CL does not exist in nature, as it is achieved with artificial light [13] . Here, nevertheless, for the first time since its discovery nearly half a century ago [40] , the CL tolerance present in wild tomato species was used for research and tested in practice. It was found that the CAB-13 gene is a key component of the CL tolerance found in wild tomato species. It was also shown that CL influences carbohydrate metabolism and photosynthesis, yet plant development and fruit set are unaffected. Finally, our results show that the concept of increasing tomato yield using this trait and CL is feasible. Genetic ( Fig. 1 ), gene expression ( Supplementary Table 3 ), silencing ( Fig. 2 ) and sequence data ( Fig. 2 and Supplementary Table 2 ) all point to the CAB-13 gene as responsible for CL tolerance in wild tomatoes, hypothetically, as a result of two copies of GT-1 consensus in its promoter. CAB-13 , a type III LHCB, belongs to the LHC supergene family. In Arabidopsis , this supergene family encodes six very similar proteins (LHCB1-6) (ref. 41 ). Tomato CAB-13 gene is homologous to Arabidopsis LHCB3 . In Arabidopsis , LHCB1–3 form the ‘major’ trimeric LHCII antenna complexes, and LHCB4–6 form the monomeric ‘minor’ antenna complexes [42] . The antenna complexes harvest light and transfer the energy to the PSII core; together they constitute the PSII–LHCII supercomplex (see ref. 43 for a recent review). In Arabidopsis , absence of LHCB3 results in alterations of the composition, structure, stability and efficiency of PSII–LHCII supercomplexes [42] , [44] , [45] , [46] . For instance, LHCB3 can be replaced by LHCB1 and/or LHCB2, but the resulting LHCII trimer binds to the PSII–LHCII supercomplex in a slightly altered position [44] . In knockout plants lacking LHCB3 (ko Lhcb3 ), the PSII–LHCII supercomplex stability is compromised in such a way that it lacks some LHCII subunits [42] . Similarly, high-light-acclimated plants show a reduction in LHCB3, which leads to higher PSII quantum yield of charge separation and supercomplexes lacking the same subunits as in ko Lhcb3 plants [45] , [46] . Here, we have shown that CL induces downregulation of tomato CAB-13 , and that CL exposure results in higher CAB-13 expression in CL-tolerant plants than in CL-sensitive plants ( Supplementary Table 3 ). This suggests that CL alters CAB-13 levels and PSII–LHCII supercomplex structure. The absorption spectra and quantum efficiencies of PSI and PSII are different, yet they work in series. For maximum efficiency, balanced excitation of PSI and PSII is vital. In response to short-term changes in light intensity and quality, LHCII trimers can move between PSI and PSII in order to keep both photosystems equally excited—a process that requires LHCII trimer phosphorylation and is known as state transitions [47] . After long-term acclimation to natural light conditions, ‘extra’ LHCII trimers (composed by LHCB1–2) are associated with both PSII and PSI; the formation of PSI–LHCII complexes appears to be required for balanced excitation of both photosystems in the long term [48] . Interestingly, in ko Lhcb3 leaves, the rate of state transitions (LHCII from PSII to PSI direction) is enhanced and the level of LHCII trimer phosphorylation is higher, suggesting that LHCB3 modulates the rate of state transitions [44] . Considering that LHCII phosphorylation and LHCB expression are possibly co-regulated [49] , the true importance and function of LHCB3 might be more than what our current knowledge suggests. The GO terms ‘chlorophyll binding’ and ‘PSI reaction centre’ were significantly enriched when A131 plants are exposed to CL, thus suggesting that the CL-induced injury in tomato might be the result of unbalanced excitation of PSI and PSII. Deletion of the GT-1 consensus binding site in CL-sensitive lines ( Fig. 2 ) suggests a connection between the CL-induced injury and light signalling. GT-1 binding sites are present in many light-regulated genes like LHC proteins (also known as Cab), the small subunit of Rubisco (RbcS) and phytochrome A [31] . Upon Ca 2+ -dependent phosphorylation, GT-1 transcription factor binds to the DNA sequence [31] , [50] , [51] . GT-1 binding sites are often found in tandem [31] . For instance, the pea RbcS-3A promoter contains six GT-1 binding sites [52] , yet a −166 deletion shows that the presence of only two of them, named boxII and boxIII, is sufficient for transcription [53] . Early studies suggested that both boxII (−150, positive strand) and boxIII (−124, negative strand) are needed for expression [54] ; however, it was later shown that instead of the core GT-1 binding site of boxIII, a GATA motif partially overlapping with boxIII is absolutely required for transcription, together with boxII [55] . Interestingly, the tomato CAB-13 promoter in CL-tolerant tomatoes shows some similarities with the pea RbcS-3A promoter; it contains a GT-1 binding site at −50 (positive strand) and another one, partially overlapped with a GATA motif, at −105 (negative strand) ( Fig. 2 ). Hence, the missing GT-1 binding site at −50 in all CL-sensitive tomato lines could be responsible for the lower expression of CAB-13 in CL-sensitive lines under CL ( Supplementary Fig. 1 and Supplementary Table 6 ). Although the GT-1 binding site of boxII and the GATA motif of boxIII are sufficient for pea RbcS-3A expression in mature leaves, sequences upstream of −170, which contain redundant GT-1 binding sites, are required for high-level expression in young developing leaves [54] . Considering that only young tomato leaves are sensitive to CL [20] , [56] , CAB-13 expression in developing tomato leaves exposed to CL might be affected by the absence of the GT-1 binding site. All together, we propose a hypothesis in which the absence of GT-1 binding site in the CAB-13 promoter allows a CL-induced downregulation of CAB-13 in developing tomato leaves, resulting, as discussed above, in unbalanced PSI and PSII excitation. Hyperaccumulation of carbohydrates, observed in CL-exposed leaves, has been proposed to induce injury in tomato plants [1] , [7] , [13] , [16] . Here, GO analysis showed that CL affects carbohydrate metabolism in uninjured leaves ( Figs 3 and 4 ). Leaf carbohydrate quantification shows that glucose and fructose concentrations are higher in CL-tolerant (CLT) than in CL-sensitive (A131) tomato plants when grown under 16-h photoperiod, and in both genotypes CL decreases glucose and fructose content. No interaction between genotype and photoperiod was observed. Interestingly, when grown under CL, sucrose content is constantly high in both genotypes ( Supplementary Table 7 ); in other words, sucrose accumulation occurs in both CLT and CL-sensitive A131 plants. If sugars play a role in inducing injury and/or downregulating photosynthesis under CL, these observations suggest that CL tolerance in CLT tomatoes is downstream carbohydrate accumulation. A recent study suggested that the tomato sugar partitioning affecting protein, a DnaJ chaperone-related protein, mediates sink–source relationships by increasing the leaf capacity to export sugars [57] . In our RNAseq data set, CL slightly downregulated sugar partitioning affecting (Solyc04g081320.2) expression (logFC=−1.057, false discovery rate (FDR) P -value=0.002) in A131 plants, yet no effect was found between A131 and CLT tomato plants under CL (FDR P -value=0.066) (see Supplementary Data 1 ). Regarding a potential application of CL tolerance, it was shown that the trait can easily be introgressed into domesticated tomato with various genetic backgrounds (A131, M82, Moneyberg, Idooll and Westland) using several wild donors ( Solanum neorickii , Solanum pennellii, Solanum habrochaites and Solanum chilense ). In addition, the yield trial has shown that tomato yield per m 2 can be increased using CL-tolerant tomato lines, up to 20% ( Fig. 7 ). Such yield increase agrees with the crop model computations, which predicted that the theoretical maximum yield increase achievable by cultivating tomatoes under CL is 22% when applying a similar photoperiod increase [23] . Nonetheless, this simulation study assumed no crop adaptations to CL, but we have observed some adaptations that could have a significant impact on yield. For instance, day respiration was higher in the tolerant genotype ( Table 1 ) and leaves were smaller when exposed to CL ( Fig. 5f ) which negatively influences light interception. Further increasing crop density could solve this and, predictable, could further increase yield under CL. Understanding why CL increases yield is a question of much interest. However, the yield trial was not designed to answer this question but rather to succeed in cultivating tomatoes under CL for the first time. Nonetheless, the results suggest that the observed yield increase was achieved by a combination of higher crop density, which was only made possible by the use of CL, and ‘night’ photosynthesis ( Supplementary Fig. 3a ); however, unquantifiable, at least in this study, contributions of other factors, like altered canopy structure ( Fig. 5 ), higher day respiration in CLTs ( Table 1 ) and unknown, yet potential, effects on assimilate partitioning and leaf senescence, prevent us from assigning a numeric contribution of each factor to the observed yield increase. Although the involvement of other genes in the CLT locus ( Fig. 1 ) cannot be completely discarded with the evidence presented here, multilevel evidence presented in this study supports the involvement of CAB-13 in this trait. This implies that photosynthesis and the PSII antenna are involved in the CL-induced injury at a higher degree than previously thought. Nonetheless, the role of carbohydrate metabolism, light signalling and the circadian clock cannot be ruled out. The identification of wild tomato CAB-13 as responsible for the CL tolerance is a significant breakthrough, and it is the base of further research on photosynthesis and its interaction with carbohydrate metabolism, light signalling and the circadian clock. Plant materials and genetic stocks All tomato ( S. lycopersicum ) varieties as well as introgression line populations and wild tomato species used in this study were provided by Monsanto Holland B.V. (Bergschenhoek, The Netherlands) with the exception of Sub-Arctic Plenty, of which seeds came from Thompson & Morgan (Ipswich, Suffolk, UK). IL from three populations were used to map the CL tolerance trait. The first IL population is a BC 3 F 3 S. neorickii (LA2133) × S. lycopersicum A131 consisting of 43 lines. This population was originally developed and described by ref. 58 . The original BC 2 F 5 S. neorickii (LA2133) × S. lycopersicum E6203 population was backcrossed with the inbred line A131 to obtain the BC 3 F 3 population that was used in this study. In this IL population, the S. neorickii chromosomes are reasonable well represented; only the bottom of chromosome 1 and 8 and the top of chromosome 11 are not presented in the population. The ‘CLT’ line used in the RNAseq experiment belongs to this population. The second population is a S. chilense (LA1959) × S. lycopersicum Moneyberg consisting of 49 lines. The population consists for 2/3 of BC 4 F 3 and 1/3 of BC 4 F 4 lines. The S. chilense chromosomes are well represented in the IL population except for the top of chromosome 5 and 6. The third IL population is a BC 3 F 4 S. pennellii (LA0716) × S. lycopersicum M82 consisting of 49 lines of which only five lines with an introgression on chromosome 7 were used. This population was developed and described by ref. 59 . For the yield trial, several CL-tolerant IL were backcrossed with the parents of ‘Idooll’ or ‘Westland’ F 1 commercial hybrids (Monsanto Holland B.V.). The wild donors of CL tolerance in those IL were S. habrochaites (lines hir135 and hir345) and S. pennellii (line pen5940). After 3–4 backcrosses, the newly bred parents, segregating as CL tolerant or sensitive, were used to generate homozygous or heterozygous and tolerant or sensitive Idooll and Westland F 1 hybrids. Genotyping IL IL were genotyped with 384 SNP markers using a custom GoldenGate genotyping assay (Illumina, San Diego, California, USA). The sequences, alleles, accession numbers and positions of the 27 SNP markers that mapped to chromosome 7 can be found in Supplementary Table 8 . Genomic marker positions were based on the public tomato reference genome v2.40 (ref. 24 ). Growth conditions and treatments For phenotyping CL tolerance of tomato varieties, introgression line populations and wild tomato species, plants were grown in climate cells at Monsanto Holland B.V. (Bergschenhoek, The Netherlands). Plants, at least four repetitions, were sown in rockwool, irrigated with hydroponic nutrient solution and grown at 21 °C and 70% RH. After growing the plants for 2 weeks under fluorescent tubes at an intensity of 120 μmol m −2 s −1 under 16-h photoperiod, plants were exposed to CL at an intensity of 120 μmol m −2 s −1 provided by high-pressure sodium (HPS) lamps. A genotype was called CL sensitive if all replicates ( n =6) showed interveinal, mottled chlorosis in young, fully expanded leaves. A genotype was called CL tolerant if the entire foliage of all replicates ( n =6) showed neither signs of chlorosis nor necrosis after at least 6 weeks of exposure to CL. Plants used for the RNAseq analysis and VIGS experiments were grown in climate cells at Wageningen University (Wageningen, The Netherlands). Plants were sown in rockwool, irrigated with hydroponic nutrient solution and grown at 21 °C and 70% RH. Light was provided by HPS lamps (Master SON-T Green Power 400 W, Philips, Eindhoven, The Netherlands) and supplemented with incandescence lamps (Philinea T30 120 W, Philips) at an irradiance of 350 μmol m −2 s −1 ; red-to-far-red ratio was 2.873, and the phytochrome photostationary state [60] was 0.857. After growing the plants for 4 weeks under 16-h photoperiod, plants were exposed to CL by leaving the lamps (HPS and incandescent) continuously ON without changing any other setting. RNAseq and GO enrichment analyses One-month-old A131 and CLT plants were transferred to CL. After 1 week of treatment, the leaflets of the topmost fully expanded leaf (fifth true leaf) were harvested for sequencing the transcriptome using SOLiD3 technology (Applied Biosystems, Foster City, California, USA). The raw reads were mapped to the public tomato genome v2.40 (ref. 24 ), using the ITAG gene annotations v2.3 and the CLC Genomics software v5.1.6 (CLCbio, Aarhus, Denmark). Further analysis was performed in R (ref. 61 ) exclusively using reads that mapped to a single place in the genome. To find differentially expressed genes the R package ‘edgeR’ was used [62] . Only genes with an expression higher than 0.01 counts per million in at least three samples were used for further analysis. A trimmed mean of M -values normalization procedure accounted for library size [63] . A generalized linear model procedure of ‘edgeR’ tested for differentially expressed genes in the contrasts A131 CL versus A131 16h and A131 CL versus CLT CL. Genes were called differentially expressed when its FDR-corrected P -value was lower than 0.05. The R package ‘GOseq’ was used for GO enrichment analysis [64] . First, the GOseq procedure calculated the probability that a gene was called differentially expressed as a function of its length; this probability was then included into the statistical model. This prevents that a GO category is called significantly enriched if contains an above-average number of long or short genes. The most accurate ‘sampling method’, included in GOseq, tested each GO category. GO categories containing less than three genes were filtered out. A GO category was called significantly enriched when its FDR-corrected P -value was lower than 0.05. The results were visualized using the R package ‘REVIGO’ [38] . VIGS RNA was extracted from a 3-week-old CLT tomato plant according to ref. 65 and purified with silica membranes columns. In short, 50 mg of frozen pulverized leaf tissue was homogenized with 500 μl of extraction buffer (350 mM glycine, 48 mM NaOH, 340 mM NaCl, 40 mM EDTA and 4% SDS) at 50 °C. Then the homogenate was extracted three times with phenol/chloroform/isoamyl alcohol (25:24:1 v/v), and later RNA was precipitated with 120 μl of 8 M LiCl. After washing the RNA with 500 μl of ethanol 70% (v/v) at −20 °C, RNA was dissolved in 87.5 μl of RNA-free water. Finally, the RNA was purified with RNeasy spin columns (Qiagen, Venlo, Netherlands). cDNA was synthesized with iScript (Bio-Rad, Hercules, California, USA) and PCR amplified using high fidelity polymerase (Invitrogen, Carlsbad, California, USA) with the primers 5′-ATTCTAGCAGTATTGGG-3′ and 5′-TCTTCCGTTCTTGATTTCCT-3′. The resulting 189-pb Lhcb3 fragment was found to be unique after blasting its sequence to the reference tomato genome. This fragment was cloned into pCR4Tm4Blunt TOPO plasmid (Invitrogen), and competent Escherichia coli (DH5αTM-T1R) cells (Invitrogen) were transformed and grown on agar plates with kanamycin (10 mg ml −1 ). The plasmid was digested with EcoRI, and the fragment cloned into EcoRI-linearized pTRV2 VIGS vector [27] , [28] ; then DH5α cells were transformed by electroporation and selected with kanamycin. After confirming fragment and plasmid integrity by sequencing and restriction analysis (XcmI and EcoRI), respectively, the pTRV2::Lhcb3 plasmid was cloned into Agrobacterium tumefaciens strain pCH32-C58C1 by electroporation. Previously described pTRV::PDS [27] and pTRV::GUS [29] constructs were used as positive and negative controls, respectively. Agrobacterium culture containing pTRV1 was mixed with each of the pTRV2-derivate cultures at 1:1 ratio at a final O.D. 600 =0.8 and used to inoculate 10-day-old A131 and CLT tomato plants grown under 16-h photoperiod following the procedure of [66] . Two and a half weeks after infiltration, pTRV2::PDS-treated plants showed photobleaching symptoms. At that point, chlorophyll fluorescence images were taken and the CL treatment started. After 3 weeks of treatment, chlorophyll fluorescence images were once more taken on the topmost fully expanded leaves. Rt–qPCR RNA and cDNA were extracted and synthesized, respectively, as described before, but treating the RNA with DNase (Sigma). The Rt–qPCR primers for Lhcb3 were 5′-CTGCTCAAACTCCTTCATACTT-3′ and 5′-AAAGGCCTCGGGATCAGC-3′. From the RNAseq data, five genes with the most stable expression across genotypes and photoperiod treatments were selected as reference genes. The used primers and genes were 5′-GCCACTTCTCCTATCAGTTTTT-3′ and 5′-CCAAAGATGAACCCCAAAACA-3′ for Solyc03g097870.2, 5′-TGGTGCTCCCCTTCCAGC-3′ and 5′-TGGCTCTCCTCCTCCGTT-3′ for Solyc06g048410.2, 5′-ATGCCTACTCGTTACACACT-3′ and 5′-CCGGTCTTGAACCTCTCCT-3′ for Solyc06g073300.1, 5′-TTCACTGCGTGTCTTCCT-3′ and 5′-CATCTTGCTTCTCACCCTT-3′ for Solyc09g010440.2, and 5′-AAACACCAAAGACGACCTCA-3′ and 5′-CACAGACAGAACGAGATCC-3′ for Solyc12g010060.1. The geometric mean of all five genes was used to normalize Lhcb3 expression. Sequencing and sequence alignment The reference tomato genome sequence v2.4 (Heinz) and the draft S. pimpinellifolium genomic scaffold sequences are publicly available [24] . The CLT locus sequence of tomato and wild tomato lines were obtained and aligned by the 150 tomato genome consortium in collaboration with the user community [25] . For A131 and CLT lines, transcriptome sequences were available from the RNAseq experiment. Lhcb3 promoter sequences from selected tomato and wild tomato lines were obtained by Sanger sequencing, using the primers 5′-TGGTGCGCATGAGTCTAAACA-3′ and 5′-CCAGCAGTATCCCATCCGTAAT-3′. CLC Workbench software v6.8.4 (CLCbio) was used for sequence alignment. Chlorophyll fluorescence imaging Intact leaflets (attached to the plant) were dark-adapted using dark adapting clips (Li-Cor Biosciences, Lincoln, USA). After 20 min of dark adaptation, leaflets were detached and immediately used for measurements in a chlorophyll fluorescence imaging system (FluorCam, Photon System Instruments, Brno, Czech Republic). FluorCam model 700MF was used in the RNAseq experiment; in the VIGS experiment, Fluorcam 800MF was used instead. Fluorcam v.5.0 and 7.0 softwares were used to control and process the images in FluorCam 700MF and Fluorcam 800MF, respectively. In both FluorCam models, maximum quantum efficiency of photosystem II ( F v /F m ) [26] was calculated following a custom-made protocol. During a period of 5 s, red–orange light-emitting diodes produced measuring light flashes (the average irradiance produced by the measuring light flashes was <0.5 μmol m −2 s −1 ); then a halogen lamp (FluorCam 700MF) or red–orange light-emitting diodes (FluorCam 800MF) produced a 1 s saturating light pulse. The saturating light pulses had an intensity of 2,500 and 3,500 μmol m −2 s −1 in Fluorcam 700MF and Fluorcam 800MF, respectively. In FluorCam 700MF, F o and F m images were recorded every 80 or 400 ms, respectively; in Fluorcam 800MF, both F o and F m images were recorded every 100 ms. Fluorescence images recorded during the first 5 s were averaged to produce a single F o image, and images recorded during the latter 1-second saturating light pulse were averaged to produce a single F m image. From these two images, a spatially resolved F v /F m image was constructed using the expression F v = F m −F o . Leaflet average F v /F m was calculated using ImageJ software version 1.44o (ref. 67 ). Yield trial The yield trial was performed on two contiguous, independent greenhouse compartments on GreenQ facilities (Bleiswijk, The Netherlands) (+52° 1′ 49.05″, +4° 31′ 46.91″). Each greenhouse compartments had six gutters, and the planted area was 124.71 and 107.76 m 2 . All plants were grafted on Maxifort (Monsanto Holland B.V., Bergschenhoek, The Netherlands) and planted according to a completely randomized block design, consisting of four blocks. To account for a potential edge effect, plants too close to the greenhouse wall were not used for any measurement. Within each block, parcels had three plants, and each plant had two stems; the resulting densities of 2.10 and 2.45 stems per m 2 was achieved by adding extra plants on the edges when needed. The crop was trained according to the high-wire system and irrigated with hydroponic nutrient solution according to standard practices. CO 2 enrichment was used with a set point of 700 p.p.m. Bumblebees (Koppert Biological Systems, Berkel en Rodenrijs, The Netherlands) were used for pollination; hive exits were open only between sunrise and sunset—bumblebees cannot navigate without the sun, yet they exit the hive if lamps are on. Leaf and fruit pruning was applied when needed to keep the vegetative and generative strength equally balanced in all F 1 lines. Temperature was adjusted weekly accordingly to crop development. As Dutch law prohibits opening the greenhouse screens before midnight when the lamps are ON [68] , the coldest period in the CL compartment was shifted to start just after midnight; the compartment at 16-h photoperiod was managed according to standard practices. The yield trial started on the 1 October 2012 with grafted plants bearing two stems and the first flower. Photoperiod was gradually increased to 16 and 24 h of light per day, reaching the final set points on the 22 and 28 November 2012, respectively. To achieve these photoperiods, HPS lamps, with an installed capacity of ±130 μmol m −2 s −1 , were used as many hours as needed; lamps were turned OFF when incoming solar irradiance was higher than 350 W m −2 . On week 5, 2013, stem density was increased to 3.15 and 3.68 stems m −2 . The trial was finalized on the 22 April 2013. Yield per F 1 hybrid line and per plot was recorded weekly. In addition, two F 1 Idooll lines were selected for performing detailed developmental and photosynthetic measurements. These lines were selected because its parents were backcrossed the most (four times). Both lines had S. pennellii as wild donor (line pen5940); one line was homozygous CL sensitive and the other one was homozygous CL tolerant. Developmental measurements were performed weekly, and they consisted of measuring leaf and stem length, recording flowering, setting and harvested truss number and keeping record of fruit set and truss load. Photosynthetic measurements were done on week 3, 2013 on the topmost fully expanded leaf. By this time, the complete canopy had developed under the 16-h photoperiod or CL. Photosynthesis measurements Photosynthesis measurements were done with a gas exchange system (LI-6400, Li-Cor Biosciences). All measurements were performed with a block temperature of 21 °C. For continuously measuring photosynthesis during two day/night cycles, the standard 2 × 3 cm chamber with a clear window (Propafilm film) was used. Greenhouse air was first buffered in a 40 l container, and then used in the measurements without further conditioning. Flow rate was set at 350 μmol air per second. IRGAs where automatically matched every 30 min and data were logged every minute. Light intensity inside the leaf chamber was estimated using the readings from the quantum sensor placed outside the chamber (LI-190, Li-Cor Biosciences) corrected with the measured light transmittance of the Propafilm film. After 2 days of measurements, the enclosed leaves expanded beyond the initial 6 cm 2 . To correct for this change in leaf area, the leaf was detached, cut and photographed at the end of the measurements. The new area was calculated using ImageJ software version 1.44o (ref. 67 ). A linear change in leaf area was assumed and used to correct all gas exchange measurements. For measuring light and CO 2 response curves, a 2 cm 2 leaf chamber equipped with a fluorometer was used (6400-40, Li-Cor Biosciences). At every change in light or CO 2 , the IRGAs where matched and chlorophyll fluorescence and gas exchange data were simultaneously logged. After dark-adapting the leaf for 20 min, F v / F m was measured. Then, waiting 5 min after each change, a 12-step light curve (20, 40, 60, 80, 100, 250, 500, 750, 1,000, 1,250, 1,500 and 1,750 μmol m −2 s −1 ) was performed at a CO 2 concentration of 600 p.p.m. ; below 100 μmol m −2 s −1 , only red light was used (restriction of the apparatus), and from 250 μmol m −2 s −1 on, red light was supplemented with 10% blue light. Finally, waiting 3 min after each change, a 9-step CO 2 curve (50, 100, 200, 300, 400, 600, 800, 1,000, 1,200 p.p.m.) was performed at a light intensity of 1,750 μmol m −2 s −1 . When necessary, water vapour was scrubbed from the greenhouse air before the injection into the leaf chamber to prevent water condensation on the IRGAs lenses. Depending on the photosynthesis rate at each CO 2 and light level, flow rate was carefully set between 200 and 300 μmol of air per second; during all measurements the flow rate was low enough to achieve a good signal-to-noise ratio (ΔCO 2 >0.2 μmol CO 2 mol −1 in 96.8% of the measurements) and, yet high enough to prevent CO 2 depletion in the leaf chamber (ΔCO 2 <30 μmol CO 2 mol −1 ) and also to reduce diffusion leaks at the minimum. In addition, all measurements were corrected for diffusion leaks using a leak rate constant calculated according to manufacturer instructions. The parameters of the FvCB model [39] , were estimated combining gas exchange and chlorophyll fluorescence data according to ref. 69 , with some modifications (see Supplementary Methods for details). Statistical analysis The observed against expected proportion in segregating F 2 population was tested with a X 2 test. Statistical significance of the leaflet average F v /F m and yield data was determined with an analysis of variance test. For the F v /F m data, a power transformation was used to achieve homogeneous variances. Analysis of variance and X 2 tests were performed with IBM SPSS Statistics software version 19 (IBM, Somers, USA). The FvCB model parameters were estimated in Microsoft Excel using the GRG nonlinear iteration procedure. How to cite this article : Velez-Ramirez, A. I. et al . A single locus confers tolerance to continuous light and allows substantial yield increase in tomato. Nat. Commun. 5:4549 doi: 10.1038/ncomms5549 (2014). Accession codes : RNAseq data generated in this study have been deposited in the NCBI Sequence Read Archive (SRA) under accession code SRP041241 .